A graphene quantum dot photodynamic therapy agent with high singlet oxygen generation Clinical applications of current photodynamic therapy (PDT) agents are often limited by their low singlet oxygen ( 1 O 2 ) quantum yields, as well as by photobleaching and poor biocompatibility. Here we present a new PDT agent based on graphene quantum dots (GQDs) that can produce 1 O 2 via a multistate sensitization process, resulting in a quantum yield of ~1.3, the highest reported for PDT agents. The GQDs also exhibit a broad absorption band spanning the UV region and the entire visible region and a strong deep-red emission. Through in vitro and in vivo studies, we demonstrate that GQDs can be used as PDT agents, simultaneously allowing imaging and providing a highly efficient cancer therapy. The present work may lead to a new generation of carbon-based nanomaterial PDT agents with overall performance superior to conventional agents in terms of 1 O 2 quantum yield, water dispersibility, photo- and pH-stability, and biocompatibility. Owing to the high mortality rate caused by malignant tumours, much effort has been devoted to identify an efficient approach to treat cancer [1] . Among the emerging cancer therapy methods, photodynamic therapy (PDT) surpasses the traditional methods (surgery, chemotherapy and radiotherapy) because it is noninvasive in nature, has fewer side effects, causes negligible drug resistance and has low systemic toxicity [2] , [3] , [4] . In PDT, cancerous cells are locally killed by reactive oxygen species (ROS) such as 1 O 2 produced by a photosensitizer (PS) under illumination and in the presence of oxygen [2] . Activatable photosensitizers, such as porphyrin, phthalocyanines and bacteriochlorin derivatives, have been demonstrated to possess simultaneous cancer imaging and therapy capabilities, and some of these photosensitizers have been approved for clinical use [5] . However, the current applications are often limited by the drawbacks of these organic PDT agents, including poor water dispersibility, photostability and their inability to be absorbed in the region (>700 nm) where the skin is most transparent [6] , [7] . Although the alternative semiconductor quantum dots (QDs) are superior to organic photosensitizers in terms of photostability and water dispersability [8] , [9] , [10] , the clinical translation of these agents has been impeded owing to their cytotoxicity and low ROS-generation efficiency [11] , [12] , [13] , [14] , [15] . Therefore, approaches such as modifying semiconductor QDs with a traditional PDT agent (porphyrin derivative, Ce6) and then coating them with a shell of peptides have been developed to reduce the cytotoxicity of these agents [16] . A PDT agent with a high 1 O 2 quantum yield and excellent photostability and biocompatibility is highly desirable. Carbon nanostructures have a wide variety of promising applications in environmental, energy and biomedical fields [17] , [18] , [19] , [20] , [21] . In particular, the photoluminescence (PL) effect of carbon QDs (CQDs) enables them to be extensively applied in bioimaging and biosensing [22] , [23] , [24] , [25] . Green-light-emitting CQDs have been conjugated to Ce6 to improve their biocompatibility and light-emission intensity [26] . This composite allowed simultaneous imaging and in vivo PDT of tumours, however, the PDT efficiency was dominated by Ce6. Very recently, it was reported that graphene quantum dot (GQDs) passivated with polyethylene glycol derivatives could generate 1 O 2 upon irradiation with blue light [27] . However, the system exhibited only limited in vitro PDT efficiency owing to a low 1 O 2 quantum yield. In this study, we prepare highly water-dispersible GQDs in large quantities using a hydrothermal method with polythiophene derivatives (PT2) as the carbon source [28] . The GQDs exhibit a broad absorption in the UV-visible region and a strong emission peaking at 680 nm. We demonstrate that the GQDs exhibit good biocompatibility and excellent 1 O 2 generation capability with a quantum yield of ~1.3. Moreover, in vitro and in vivo studies suggest that the GQDs can be applied as a PDT agent for the simultaneous imaging and highly efficient treatment of cancer. Structure and composition of GQDs To investigate the intrinsic crystal structure of GQDs, scanning transmission electron microscopy (STEM) was performed. 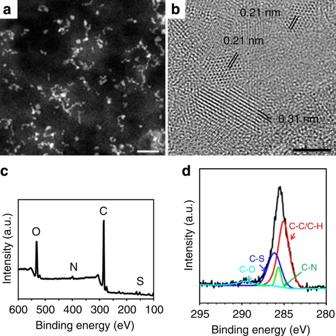Figure 1: Characterization of GQDs. (a) TEM images. Scale bar, 20 nm. (b) HRTEM images. Scale bar, 2 nm. (c) XPS survey spectrum. (d) Deconvolution of high-resolution C1s XPS spectra. Figure 1a presents a STEM image of the GQDs, with diameters ranging from 2 to 6 nm. The high-resolution TEM (HRTEM) observation of the GQDs in Fig. 1b reveals the crystallinity of the GQDs; the labelled interplanar distance of 0.21 nm agrees with the (100) lattice spacing of graphene along the [001] direction, and that of 0.31 nm corresponds to the lattice fringes of (002) planes [29] , [30] . A typical X-ray diffraction pattern and a Raman spectrum ( Supplementary Fig. 1 ) further verify the sp 2 configuration of the GQDs [31] , [32] . X-ray photoelectron spectroscopy (XPS) measurements were performed to probe the composition of the GQDs. The survey spectrum in Fig. 1b indicates the presence of carbon, nitrogen, sulphur and oxygen; deconvolution of the high-resolution C1s XPS spectra ( Fig. 1c ) reveals peaks at 285.0, 285.7, 286.2 and 289.7 eV, corresponding to C–C, C–N, C–S and C–O bonding, respectively. The nitrogen and sulphur content were evaluated to be 1.6% and 5.8%, respectively ( Supplementary Fig. 2a ). The high-resolution N1s and S2p spectra in Supplementary Fig. 2b,c also support the formation of C–N and C–S bonding, which implies the incorporation of nitrogen and sulphur into the GQDs. Moreover, oxygen is physically and chemically adsorbed on the GQDs ( Supplementary Fig. 2d,e ). Figure 1: Characterization of GQDs. ( a ) TEM images. Scale bar, 20 nm. ( b ) HRTEM images. Scale bar, 2 nm. ( c ) XPS survey spectrum. ( d ) Deconvolution of high-resolution C1s XPS spectra. 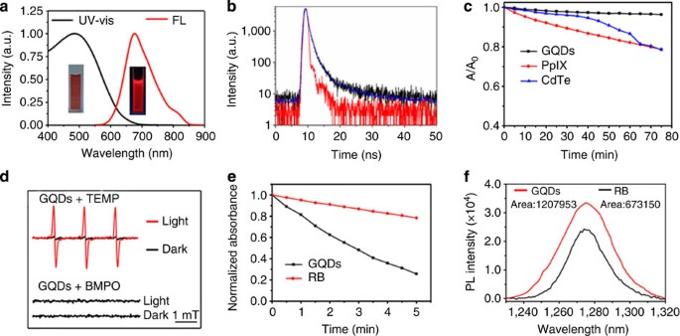Figure 2: Photophysical and photochemical properties of GQDs. (a) Normalized UV–vis absorption and emission spectra (λex=500 nm) of the GQDs dispersed in water at room temperature. The inserts show a photograph and fluorescence image of the GQD solution under UV light (365 nm). (b) Fluorescence decay curve (black line) of GQDs recorded at 680 nm with an excitation of 488 nm. Red line: the instrument noise; blue line: fitting of the fluorescence decay curve. Fit=A+B1exp(−t/τ1)+B2exp(−t/τ2)+B3exp(−t/τ3;τ1=0.27 ns,τ2=1.10 ns,τ3=7.52 ns). (c) A comparison of the photostabilities of the GQDs, CdTe QDs and PpIX. All of the samples were continuously irradiated using a 500-W xenon lamp. A0and A are the absorbance of the samples at 470 nm before and after irradiation, respectively. After 75 min of irradiation, no obvious decline was observed in the absorbance of the GQDs, while the absorbance of PpIX and the CdTe QDs decreased below 78% of their initial value. (d) The ESR signals of1O2(up) and other ROS (down) obtained upon irradiation of GQDs for 8 min in the presence of 2,2,6,6-Tetramethylpiperidine and 5-tert-butoxycarbonyl 5-methyl-1-pyrrolineN-oxide, respectively. (e) The normalized absorbance of Na2-ADPA at 378 nm as a function of irradiation time in the presence of GQDs and RB. (f) The1O2emissions at ~1,280 nm induced by the GQDs and RB in a CH3CN-D2O mixture solution (v/v=15/1) under excitation with a 532-nm laser. Full size image Photophysical and photochemical properties of GQDs Figure 2a presents the UV–vis absorption and PL spectra of the GQDs, illustrating that the GQDs have a broad absorption, from 400 to 700 nm, and a deep-red emission peaking at 680 nm. The GQDs exhibited a large Stokes shift of 205 nm, implying that the self-absorption of their emission and the measurement interference between excitation light and scattered light could be minimized. To further understand the luminescence properties, the time-resolved PL spectra of GQD aqueous solution were measured with an excitation of 488 nm. Analysis of the fluorescence decay kinetics revealed three exponential decays, with the longest lifetime being 7.52 ns ( Fig. 2b ); a lifetime on the ns level suggests the singlet state nature of the GQD emission. The fluorescence quantum yield of the GQDs was measured to be 0.054 in an O 2 atmosphere using a spectrometer attached to an integrating sphere. Both the fluorescence lifetime and fluorescence quantum yield of the GQDs increased when the measurements were performed in an air or N 2 atmosphere. A similar tendency was also observed in 9,10-dicyanoanthracene, which contains a fused-ring aromatic with a large π-conjugated structure and enables 1 O 2 generation from both singlet and triplet states ( Supplementary Table 1 ) [33] . Furthermore, the GQDs exhibited superior photostability to CdTe QDs (conventional red-emitting semiconductor QDs) and protoporphyrin IX (PpIX, a classic photosensitizer; Fig. 2c and Supplementary Fig. 3 ) as well as good pH stability ( Supplementary Fig. 4 ), which are essential for biomedical applications [34] , [35] , [36] . Figure 2: Photophysical and photochemical properties of GQDs. ( a ) Normalized UV–vis absorption and emission spectra ( λ ex =500 nm) of the GQDs dispersed in water at room temperature. The inserts show a photograph and fluorescence image of the GQD solution under UV light (365 nm). ( b ) Fluorescence decay curve (black line) of GQDs recorded at 680 nm with an excitation of 488 nm. Red line: the instrument noise; blue line: fitting of the fluorescence decay curve. Fit=A+B 1 exp(− t / τ 1 )+B 2 exp(− t / τ 2 )+B 3 exp(− t / τ 3 ; τ 1 =0.27 ns, τ 2 =1.10 ns, τ 3 =7.52 ns). ( c ) A comparison of the photostabilities of the GQDs, CdTe QDs and PpIX. All of the samples were continuously irradiated using a 500-W xenon lamp. A 0 and A are the absorbance of the samples at 470 nm before and after irradiation, respectively. After 75 min of irradiation, no obvious decline was observed in the absorbance of the GQDs, while the absorbance of PpIX and the CdTe QDs decreased below 78% of their initial value. ( d ) The ESR signals of 1 O 2 (up) and other ROS (down) obtained upon irradiation of GQDs for 8 min in the presence of 2,2,6,6-Tetramethylpiperidine and 5-tert-butoxycarbonyl 5-methyl-1-pyrroline N -oxide, respectively. ( e ) The normalized absorbance of Na 2 -ADPA at 378 nm as a function of irradiation time in the presence of GQDs and RB. ( f ) The 1 O 2 emissions at ~1,280 nm induced by the GQDs and RB in a CH 3 CN-D 2 O mixture solution (v/v=15/1) under excitation with a 532-nm laser. Full size image The electron spin resonance (ESR) technique was employed to detect the ROS generation by the GQDs under irradiation. 2,2,6,6-Tetramethylpiperidine and 5-tert-butoxycarbonyl 5-methyl-1-pyrroline N -oxide were used as 1 O 2 and O 2 −· (or OH · ) trappers, respectively. As illustrated in Fig. 2d (top, red line) and Supplementary Fig. 5 , a characteristic 1 O 2 -induced signal, 2,2,6,6-tetramethylpiperidine-1-oxyl, was observed in the ESR spectra only under irradiation, and its intensity increased with the increase in irradiation time. No other ROS signals were observed ( Fig. 2d , bottom). These results verify that it is the energy transfer (ET), not the electron transfer, from the GQDs to oxygen that is responsible for the sensitization of ground-state oxygen 2 . To assess the ability of GQDs to generate 1 O 2 , the 1 O 2 quantum yield was measured using a chemical trapping method with disodium 9,10-anthracendipropionic acid (Na 2 -ADPA) as the trapping agent and Rose Bengal (RB) as the standard photosensitizer ( 1 O 2 quantum yield Φ RB =0.75 in water) [14] . As illustrated in Fig. 2e , in the presence of GQDs or RB under irradiation with white light, the absorbance of the Na 2 -ADPA solution at 378 nm, decreased gradually with prolonged irradiation time, indicating the degradation of Na 2 -ADPA by 1 O 2 generated by GQDs and RB [37] . Nevertheless, the degradation rate of Na 2 -ADPA resulting from the GQDs was far larger than that from the RB. Thus, the 1 O 2 quantum yield of the GQD solution was calculated to be 1.3 ( Supplementary Fig. 6 and Supplementary Note 1 ). Moreover, measurements at different excitation wavelengths, 538, 549 and 562 nm, also revealed an almost consistent 1 O 2 quantum yield of the GQDs of ~1.3 ( Supplementary Fig. 7 and Supplementary Table 2 ). By comparing the peak areas of 1 O 2 emission at ~1,280 nm induced by the GQDs and RB in a CH 3 CN-D 2 O solution under excitation with a 532-nm laser, the GQD 1 O 2 quantum yield was determined to be 1.34 based on the known value of Φ RB =0.76 in CH 3 CN, as depicted in Fig. 2f (refs 38 , 39 ). This result agrees very well with that obtained using the chemical trapping method above. 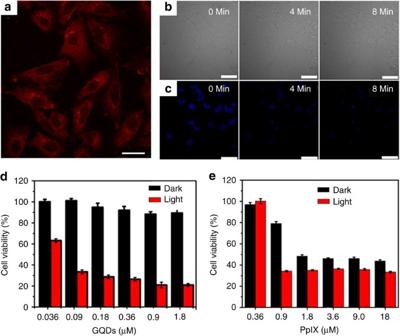Figure 3:In vitroimaging and PDT. (a) Confocal fluorescent microscopy image of HeLa cells labelled with GQDs (0.4 μM). Scale bar, 20 μm. (b) Time-dependent confocal bright field and (c) corresponding fluorescence images of HeLa cells incubated with GQDs (0.4 μM) and Hoechst 33342 (1.8 μM) after irradiation with 405 and 633 nm lasers. Scale bar, 50 μm. Dose-dependent PDT effects of the cell viability of HeLa cells: (d) GQDs in the concentration range 0.036–1.8 μM and (e) PpIX in the concentration range 0.36–18 μM. Further investigation illustrated that the 1 O 2 quantum yields were maintained at ~1.3 at pH values ranging from 6 to 8 ( Supplementary Table 3 ). To the best of our knowledge, this efficiency is the highest 1 O 2 -generating efficiency ever reported for PDT agents and is approximately twice as high as that of all of the state-of-the-art PDT agents [6] , [12] . In vitro imaging and PDT These highly photostable, water-dispersible and red-emitting GQDs can be used as fluorescence-imaging agents. Staining HeLa cells with GQDs led to strong PL emission from the cells; the corresponding fluorescence image in Fig. 3a demonstrates that the GQDs labelled only the cytoplasm and not the nucleus, similar to the observations for other C-dots [40] . Figure 3: In vitro imaging and PDT. ( a ) Confocal fluorescent microscopy image of HeLa cells labelled with GQDs (0.4 μM). Scale bar, 20 μm. ( b ) Time-dependent confocal bright field and ( c ) corresponding fluorescence images of HeLa cells incubated with GQDs (0.4 μM) and Hoechst 33342 (1.8 μM) after irradiation with 405 and 633 nm lasers. Scale bar, 50 μm. Dose-dependent PDT effects of the cell viability of HeLa cells: ( d ) GQDs in the concentration range 0.036–1.8 μM and ( e ) PpIX in the concentration range 0.36–18 μM. Full size image The photodynamic activity of the GQDs against cancer cells was investigated by monitoring the morphology variation of HeLa cells in the presence of GQDs using laser-scanning confocal microscopy. In these experiments, Hoechst 33342 was also added to stain the nucleus. As demonstrated in Fig. 3b , irradiation led to cell morphology changes, including the shrinkage of cells and the formation of numerous blebs. The corresponding fluorescence images in Fig. 3c and Supplementary Fig. 8 also confirm that photo-induced cell death was accompanied by nuclear condensation [41] , [42] . The process of cell death is also presented in two video files, which were recorded with bright-field and fluorescent microscopes ( Supplementary Movies 1 and 2 ). In control experiments, the cells did not undergo obvious morphological changes in the absence of GQDs ( Supplementary Fig. 9 ). A standard 3-(4,5-dimethylthiazol-2-yl)-2,5-diphenyl-2H-tetrazolium hydrobromide (MTT) assay was performed to quantitatively evaluate the PDT efficiency and cytotoxicity of the GQDs compared with the classic photosensitizer PpIX. In these experiments, HeLa cells were irradiated for a constant duration of 10 min in phosphate-buffered solution (PBS) with GQDs from 0.036 to 1.8 μM or PpIX from 0.36 to 18 μM, as illustrated in Fig. 3d,e , respectively. A cell viability of 60% was observed in the presence of 0.036 μM GQDs; this value decreased with increasing GQD concentration, decreasing to ~20% for the 1.8-μM GQD solution. However, GQDs have little effect on the survival of HeLa cells in the dark even at a concentration of 1.8 μM, indicating the low cytotoxicity and good biocompatibility of GQDs [23] . By contrast, a much smaller cell viability of 55% was obtained for the 1.8-μM PpIX solution in the dark condition, and more than 35% of the cells survived even upon irradiation ( Fig. 3e ). Further increasing the PpIX concentration did not induce an obvious change in cell viability. It was also observed that GQDs exhibit an even stronger PDT effect than PpIX at one-tenth the concentration. The above results verify that GQDs are superior to PpIX in terms of both their high PDT efficiency and low cytotoxicity. In vivo imaging and PDT To investigate the in vivo fluorescence imaging capability of GQDs, 20 μl GQD aqueous solution (27 μM) was injected into the back of a nude mouse. As depicted in Fig. 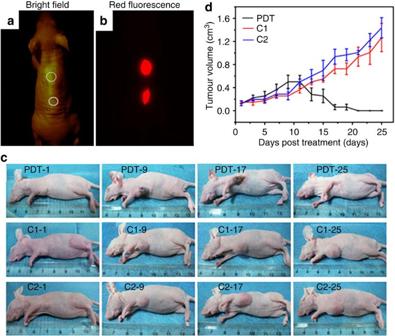Figure 4:In vivoimaging and PDT. (a) Bright-field image and (b) red-fluorescence image after subcutaneous injection of GQDs in different areas. The excitation wavelength was 502–540 nm, and the collected fluorescence channel was 695–775 nm. (c) Photographs of mice after various treatments on the 1st, 9th, 17th and 25th day. (PDT: GQDs+light irradiation; C1: GQDs only; C2: light irradiation only.) (d) Time-dependent tumour growth curves (n=5) after different treatments.P<0.05 for each group. 4a,b , the injection sites showed a much higher fluorescence intensity than the background signal produced by the mouse skin, and a high signal-to-noise ratio of 229.5 was achieved ( Supplementary Table 4 ). More importantly, no apparent fluorescence intensity decay was observed at the injection sites, and the injected GQDs did not show evidence of obvious diffusion, even 1 week after injection ( Supplementary Fig. 10 ). Figure 4: In vivo imaging and PDT. ( a ) Bright-field image and ( b ) red-fluorescence image after subcutaneous injection of GQDs in different areas. The excitation wavelength was 502–540 nm, and the collected fluorescence channel was 695–775 nm. ( c ) Photographs of mice after various treatments on the 1st, 9th, 17th and 25th day. (PDT: GQDs+light irradiation; C1: GQDs only; C2: light irradiation only.) ( d ) Time-dependent tumour growth curves ( n =5) after different treatments. P <0.05 for each group. Full size image The performance of the GQDs for in vivo PDT was evaluated using female BALB/nu mice with subcutaneous breast cancer xenografts as an animal model. Three groups of MDA MB-231 green-fluorescent protein tumour-bearing mice with 5 mice per group were used. For the PDT group, mice were intratumorally injected with GQDs (dose=4 mg kg −1 ) and then irradiated twice, on the first and seventh days, for 10 min with white light (400–800 nm) at a power density of 80 mW cm −2 . The control groups included mice that received a GQD injection at the same dose but were not irradiated (the C1 group) and mice that did not received a GQD injection but were irradiated (the C2 group). The tumour sizes were measured using a caliper every other day. As illustrated in Fig. 4c , in the PDT group, the tumours first turned dark and festered, which increased the tumour size slightly. The tumours began to decompose after 9 days and were destroyed after 17 days, leaving black scars at the original sites, which fell off ~1 week later [43] . No tumour regrowth was observed in the PDT group over the course of 50 days. In contrast, the tumours in the C1 and C2 groups grew significantly during the study period ( Fig. 4d ) and exhibited strong green fluorescence ( Supplementary Fig. 11 ), indicating that neither light irradiation nor GQD injection alone inhibited the tumour growth. Our experiments also ruled out the photothermal effect of GQDs in killing the tumour cells ( Supplementary Fig. 12 and Supplementary Note 2 ). Moreover, the in vivo toxicity of the GQDs was also roughly estimated by monitoring the weight change of the mice in the study period, and no obvious side effects were revealed ( Supplementary Fig. 13 ). In conventional PDT agents, such as porphyrin and phthalocyanines, 1 O 2 is generated by ET from the excited triplet state (T 1 ) of the sensitizer to the ground-state oxygen ( 3 O 2 ), and the 1 O 2 quantum yield is less than 1.0 ( Fig. 5a , left). The extremely high 1 O 2 quantum yield of the GQDs is considered to stem from a new 1 O 2 -generating mechanism, which can be termed multistate sensitization (MSS). According to the absorption and fluorescence spectra, the excited singlet state (S 1 ) energy of the GQDs was estimated to be ~49.3 kcal mol −1 , and the T 1 energy was estimated to be between 22.5 and 26.5 kcal mol − 1 above the ground state (G; Supplementary Fig. 14 and Supplementary Note 3 ). The energy gap (Δ E ST ) between S 1 and T 1 was thus calculated to be ~22.8~26.8 kcal mol − 1 . In this case, both Δ E ST and Δ E TG (the energy gap between T 1 and G) are larger than the formation energy of 1 O 2 (22.5 kcal mol − 1 ). Therefore, the 1 O 2 may be generated by two pathways: that is, in addition to the conventional pathway, by ET from T 1 (ET 1 in Fig. 5a and equation (1)), the ET from S 1 to 3 O 2 may also lead to 1 O 2 generation during the S 1 –T 1 intersystem crossing transition (ET 2 in Fig. 5a and equation (2)). Therefore, an overall 1 O 2 quantum yield greater than 1.0 can be achieved [33] , [44] . 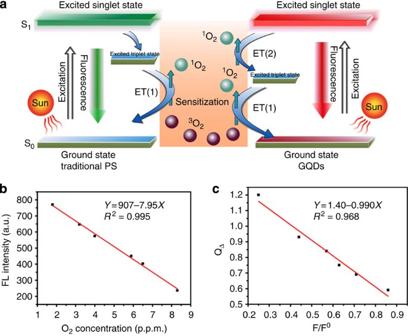Figure 5: Multistate sensitization mechanism. (a) Schematic illustration of the1O2generation mechanisms by conventional PDT agents (left) and GQDs (right). (b) Fluorescence intensity of GQDs at 680 nm versus the O2concentration in solution. (c) The dependence of the1O2quantum yield (QΔ) on the fluorescence intensity ratio at 680 nm (F/F0). Figure 5: Multistate sensitization mechanism. ( a ) Schematic illustration of the 1 O 2 generation mechanisms by conventional PDT agents (left) and GQDs (right). ( b ) Fluorescence intensity of GQDs at 680 nm versus the O 2 concentration in solution. ( c ) The dependence of the 1 O 2 quantum yield ( Q Δ ) on the fluorescence intensity ratio at 680 nm ( F / F 0 ). Full size image To further verify the MSS mechanism,we measured the fluorescence intensity at 680 nm and the 1 O 2 quantum yield of GQDs in solutions with different oxygen concentrations. Theoretically, in the MSS process, the 1 O 2 yield ( Q Δ ) can be expressed as a function of the oxygen-dependent fluorescence intensity, as described in equation (3) [44] where Q ΔM is the maximum 1 O 2 yield by ET from the S 1 and T 1 states, k is a coefficient related to the formation efficiency of T 1 and 1 O 2 yields from S 1 and T 1 states, respectively, and F 0 and F are the fluorescence intensities of GQDs at 680 nm in the absence and presence of O 2 , respectively. As illustrated in Fig. 5b , the fluorescence intensity of the GQD solution at 680 nm decreased linearly with the increase in the O 2 concentration in solution. Extrapolating the line produced the fluorescence intensity in the absence of O 2 (F 0 ): 907. On the basis of Fig. 5b , a linear dependence of Q Δ on F / F 0 was plotted, as presented in Fig. 5c . The interception of the line with the Q Δ axis yields a Q ΔM of 1.4, which coincides very well with our experimental observations. The MSS process of GQD S generating 1 O 2 was thus further verified. The MSS mechanism proposed here also suggests that a 1 O 2 quantum yield higher than 1.0 can be achieved only in the visible region (shorter than 636 nm, corresponding to the theoretical photo energy to drive the MSS for 1 O 2 generation). In summary, we have demonstrated an approach to prepare GQDs on a large scale using a simple hydrothermal method with polythiophenes as the precursors. The GQDs exhibit a combination of properties, including broad absorption from the visible to the NIR, deep-red emission, good aqueous dispersibility, high photo- and pH stability and favourable biocompatibility. More importantly, the GQDs exhibited a high 1 O 2 generation yield, greater than 1.3 (approximately twice as high as that of all of the state-of-the-art PDT agents) via a new MSS process. The collective properties of the GQDs enable them to act as a multifunctional nanoplatform for the simultaneous imaging and highly efficient in vivo PDT of cancer. Although the high 1 O 2 generation yield of GQDs was achieved only in the visible light region, there are important applications for medical treatment, such as PDT of skin cancers and tumours located near the skin. In these cases, a high 1 O 2 quantum yield is favourable. Owing to their high 1 O 2 generation efficiency, the GQDs can also be applied as efficient, environment friendly and visible-light-responsive photocatalysts for the degradation of persistent organic pollutants and microorganisms. Synthesis of PT2 PT2 was synthesized as reported recently by our group [28] , the synthetic rout can be detailed as follows and Supplementary Fig. 15 . In brief, compoud 1 was abtained by nucleophilic addition with 4-Bromobenzyl bromide and N , N -dimethyldodecylamine in a mixed solvent (CH 2 Cl 2 /CH 3 OH=3/2) under N 2 protection. Then, compoud 1 via a suzuki reaction with thiophene-3-boronic acid catalysed by Pd(PPh 3 ) 4 leads to compoud 2 . Subsequently, PT2 was prepared via an oxidative polymerization with compoud 2 under nitrogen catalysed by FeCl 3 in anhydrous CHCl 3 . Synthesis of GQDs The GQDs were prepared by hydrothermal treatment of polythiophene (PT2). In a typical synthesis, 30 mg of PT2 was dispersed in 40 ml of NaOH solution (0.5 mM). The mixture was treated ultrasonically for 30 min and then transferred into an autoclave and heated at 170 °C for a period of 24 h. After cooling to room temperature, the GQDs were collected by removing the large particles, through filtering using 0.22-μm membranes, and then dialysed against distilled water several times to remove the residual NaOH. The GQDs were dispersed in water for further characterization and use. Molecular weight measurements To calculate the molar concentration of the GQDs, we employed the gel permeation chromatography (GPC) method to evaluate their molecular weight, using polystyrene as the standard and N,N-dimethylformamide (DMF) as the eluent (GPC, Agilent 1100). The media molecular weight and weight-average molar mass ( M w) were 7.46 × 10 4 and 9.3 × 10 4 g mol −1 , respectively. The molecular weight used in the manuscript was 7.46 × 10 4 g mol −1 , the media molecular weight. 1 O 2 quantum yield measurements via the chemical method Water-soluble Na 2 -ADPA was used as the 1 O 2 -trapping agent, and RB was used as the standard photosensitizer. In the experiments, 60 μl of Na 2 -ADPA solution (1 mg ml − 1 ) was added to 1.5 ml of GQD solution, and white light (400–800 nm) with a power density of 6.5 mW cm − 2 was employed as the irradiation source. To eliminate the inner-filter effect, the absorption maxima of RB and the GQDs were adjusted to ~0.2 OD. The absorption of Na 2 -ADPA at 378 nm was recorded at various irradiation times to obtain the decay rate of the photosensitizing process. The 1 O 2 quantum yield of the GQDs in water ( Φ GQDs ) was calculated using the following formula: where K GQDs and K RB are the decomposition rate constants of Na 2 -ADPA by the GQDs and RB, respectively. A GQDs and A RB represent the light absorbed by the GQDs and RB, respectively, which are determined by integration of the optical absorption bands in the wavelength range 400–700 nm. Φ RB is the 1 O 2 quantum yield of RB, and Φ RB =0.75 in water. For the 1 O 2 quantum yield measurements at different pH values, the pH value of the GQD/Na 2 -ADPA mixture solutions was adjusted to 6.0 and 8.0 using HCl and NaOH, respectively. For the fluorescence intensities and 1 O 2 quantum yield measurements under different oxygen concentrations, the fluorescence intensities and quantum yields of 1 O 2 of the GQD solutions were determined as a function of the dissolved oxygen concentration in the range from 1.8 to 8.5 p.p.m. The oxygen concentration was varied in the following manner: the GQD solutions were deoxygenated by three freeze-pump-thaw cycles and then replenished with pure oxygen. The final concentrations of oxygen were determined using a dissolved oxygen meter (Beijing Time power Measure and Control Equipment Co., Ltd). Before each measurement of the quantum yields of 1 O 2 of the GQDs, the corresponding fluorescence spectra were detected to demarcate their fluorescence intensities, and then the 1 O 2 quantum yields of the GQDs were measured using the chemical trapping method. 1 O 2 quantum yield measurements by detecting 1 O 2 emission The 1 O 2 emission signals of the GQDs were detected in a HITACHI FL 900 fluorescence spectrophotometer with a 532-nm excitation laser and a NIR detector. Considering the short PL lifetime of 1 O 2 in water, the GQD solution was lyophilized, and the solid power was dissolved in a 15:1 (v/v) CH 3 CN-D 2 O solution. The absorptions of RB and the GQDs at 532 nm were adjusted to ~0.2 OD. The 1 O 2 quantum yield of the GQDs could be obtained using where I GQDs and I RB represent the PL peak areas of 1 O 2 produced by the GQDs and RB, respectively. Photostability evaluation of GQDs HeLa cells were obtained from the Peking Union Medical College. The HeLa cells were cultured in fresh media (DMEM/F12 supplemented with 10% fetal bovine serum, 50 unit ml −1 of penicillin, and 50 μg ml −1 of streptomycin) at 37 °C in a humidified incubator containing 5% CO 2 . The HeLa cells were incubated with 40 μl of GQDs (1 mg ml −1 ) or 40 μl of CdTe QDs (1 mg ml −1 ) in 1 ml of culture medium for 60 min at 37 °C. Then, the cells were washed using PBS and fixed with 4% paraformaldehyde in PBS for 20 min. The fixed HeLa cells were carefully washed with PBS three times. These cells were then irradiated and imaged using a Nikon C1 laser-scanning confocal microscope. The windows for the GQDs and CdTe QDs were collected at 680–740 and 580–640 nm, respectively. The images were captured with a cooled CCD camera at 100-ms intervals for each colour automatically. In vitro imaging and PDT In the in vitro imaging experiments, HeLa cells were incubated with 40 μl of GQDs (0.4 μM) in 1 ml of culture media at 37 °C. After incubating the mixtures for 1 h, the cells were washed with PBS twice to remove non-specifically bound QDs. Images were also acquired with a Nikon C1si laser scanning confocal microscopy. In the in vitro PDT experiments, HeLa cells were incubated with 20 μl of Hoechst 33342 (1.8 μM) for 20 min, and then 40 μl of GQDs (0.4 μM) were added to the culture medium for 1 h at 37 °C. The control experiments did not include GQDs. After the medium was removed, the cells were carefully washed twice with PBS. Then, the HeLa cells were continuously irradiated using 405 and 637 nm lasers equipped with scanning confocal microscopy. Images were captured with a cooled CCD camera at 100-ms intervals for each colour automatically. To compare the dark toxicity and phototoxicity of the GQDs and PpIX QDs, the GQD stock solutions were diluted with fresh medium to various concentrations (0.036, 0.09 0.18, 0.36, 0.9 and 1.8 μM). The PpIX stock solutions were also diluted with fresh medium to various concentrations (0.36, 0.9, 1.8, 3.6, 9.0 and 18 μM). The cell medium was then exchanged for different concentrations of GQDs or PpIX medium solution. The cells were then incubated with these solutions at 37 °C in 5% CO 2 for 4 h, and the cultures were then irradiated using a 500-W Xe lamp as the light source with an intensity of 6.5 mW cm −2 for 0 or 10 min before removing the GQDs or PpIX solution and adding fresh medium. Subsequently, the plates were incubated at 37 °C in 5% CO 2 for 24 h. The cell medium solutions were exchanged for 100 μl of fresh medium, followed by the addition of 20 μl of MTT solution to each well. The culture plates were then incubated at 37 °C in 5% CO 2 for 4 h. The culture medium was discarded, and 100 μl of dimethylsulfoxide was added. The absorbance of an untreated cell population under the same experimental conditions was used as the reference point to establish 100% cell viability. In vivo imaging and PDT Animal experiments were approved by the China Committee for Research and Animal Ethics in compliance with the law on experimental animals. All animal experiments were conducted at Anticancer Biotechnology (Beijing) Co. Ltd. For the in vivo imaging, female BALB/nu mice (6 weeks old, 18–20 g) received a subcutaneous injection of 20 μl (27 μM) GQD aqueous solution. The excitation wavelength was 502–540 nm, and the collected fluorescence channels were 695–775 nm. For the in vivo PDT treatment, female BALB/nu mice with subcutaneous breast cancer (MDA MB-231 green-fluorescent protein) xenografts were selected as the animal model. The in vivo fluorescence images were acquired using a FluorVivo Model-300. Photothermal effect measurements Photothermal effect data were acquired from Agilent 34970A using a T type thermocouple. White light (400–800 nm) was generated from a xenon light source (Solar-500). The intensity of the incident beam was determined by a radiometer (Photoelectric Instrument Factory of Beijing Normal University). To measure the photothermal conversion performance of the GQDs, 1.2 ml of GQD (13.5 or 27 μM) solution was introduced into a quartz cuvette and irradiated with white light (400–800 nm) at a power density of 80 mW cm −2 for 20 min. Pure water was used as a negative control. A thermocouple probe with an accuracy of 0.1 °C was inserted into the GQD aqueous solution perpendicular to the light path. The temperature was recorded at 1-s intervals by a digital thermometer with a thermocouple probe. Sample characterizations STEM and HRTEM images were recorded on a Cs-corrected Titan 80–300 microscope operated at 300 kV. X-ray diffraction patterns were obtained using an X-ray diffractometer (Bruker, Germany) with Cu-Kα radiation. The 2 θ scanning range was 10° to 80° with a scanning speed of 0.1° s −1 . XPS was performed using an ESCALAB 250 spectrometer with Al Kα X-ray excitation (1,486.6 eV). Raman spectra were measured using an Invia-Reflex Raman system using a 785-nm laser. UV–vis and fluorescence spectra were obtained using Hitachi U-3010 and F-4500 spectrophotometers, respectively. ROS were detected using the ESR technique (ESP300E, Bruker). How to cite this article: Ge, J. et al. A graphene quantum dot photodynamic therapy agent with high singlet oxygen generation. Nat. Commun. 5:4596 doi: 10.1038/ncomms5596 (2014).